Sumoylation controls the timing of Tup1-mediated transcriptional deactivation The small ubiquitin-like modifier (SUMO) is implicated in various cellular activities, including transcriptional regulation. We previously showed that the yeast activator Gcn4 becomes sumoylated during activation, facilitating its eventual promoter eviction and transcriptional shut off. Here we show that the corepressor Tup1 is sumoylated, at two specific lysines, under various stress conditions. Mutation of these sites has no effect on Tup1 recruitment or RNAP II promoter occupancy immediately following induction. However, Tup1 levels subsequently decrease, while RNAP II and transcription increase in Tup1 mutant cells. Consistent with this, a Tup1 mutant displaying increased sumoylation led to reduced transcription. We also show that coordinated sumoylation of Gcn4 and Tup1 enhances Gcn4 promoter eviction and that multiple Tup1-interacting proteins become sumoylated after stress. Together, our studies provide evidence that coordinated sumoylation of Gcn4, Tup1 and likely other factors dampens activated transcription by stabilizing Tup1 binding and stimulating Gcn4 and RNAP II removal. The small ubiquitin-like modifier (SUMO) polypeptide is present in all eukaryotes and is highly conserved from yeast to humans. SUMO covalently modifies many proteins that participate in diverse cellular processes, including transcriptional regulation, subcellular localization, DNA repair and signal transduction [1] , [2] , [3] , [4] . Many SUMO substrates are transcriptional activators, repressors, co-activators or co-repressors. Two lines of evidence have linked SUMO modifications with transcriptional repression [1] , [5] . First, in many cases interfering with sumoylation of transcriptional regulators at promoter regions leads to transcriptional activation. Second, sumoylated proteins can be recruited into repressive environments in higher eukaryotes, such as PML nuclear bodies. However, more recent studies have shown that SUMO modification of promoter-bound factors also occurs during the process of gene activation, suggesting a possible positive role in transcriptional control, in yeast [6] , [7] , [8] as well as mammalian [9] , [10] cells. Modulation of SUMO levels at gene promoters is emerging as an important aspect of transcriptional activation. For example, activation of several inducible genes in yeast caused not only accumulation of SUMO at promoter regions, but also recruitment of Ubc9, the SUMO E2 conjugating enzyme, indicating that activation involves sumoylation of promoter-bound factors. However, Ubc9 inactivation, while reducing sumoylation at the induced promoters, paradoxically resulted in increased transcription [6] and the presence of Ulp1, a SUMO protease, is important for optimal gene activation [8] . Providing an explanation for these observations, the reduced sumoylation brought about by destabilizing Ubc9 impaired the cell’s ability to shut off activated transcription appropriately, indicating that SUMO can facilitate transcriptional deactivation. Subsequently, the transcriptional activator Gcn4 was identified as one of the promoter-associated SUMO substrates, and Gcn4 sumoylation was shown to be required for its efficient removal from target promoters following RNA polymerase II (RNAP II) recruitment [7] . A similar result has also been reported for the mammalian activator AP-1 (ref. 9 ). Transcriptional activation is invariably dependent on multiple cofactors in addition to the activator. For example, for Gcn4 these include SAGA, SWI/SNF and RSC chromatin remodelling complexes, the SRB/MED complex, the transcriptional regulator CCR4-NOT and the repressive Cyc8/Tup1 complex [11] , [12] , [13] . Some of the subunits of these complexes, including, for example, Gcn5, Snf2 and Tup1, have been identified as SUMO substrates in large-scale proteomics studies [14] , [15] , [16] , [17] . However, whether sumoylation of these proteins contributes to their function in gene control, and if so how, remains mostly elusive. Tup1 has been suggested to function as both a corepressor and coactivator. The protein, which is conserved throughout eukaryotes [18] , was one of the first to be characterized as a transcriptional corepressor [19] , [20] , forming a complex with Cyc8 to mediate repression of diverse sets of genes under various stress conditions [21] . However, several studies have found that Tup1 remains associated with promoters of target genes after activation [13] , [22] , [23] . For example, Tup1 is bound to many glucose-repressed genes even after glucose repression is removed [23] . Tup1 has also been shown to play a role in recruitment of SAGA, SWI/SNF and mediator to promoters [13] , [24] , [25] , [26] . Therefore, it has been proposed that Tup1 may switch from acting as a corepressor to a coactivator during transcriptional activation [25] , [27] , [28] . Consistent with this, Tup1 binds to the ARG1 promoter after activation, and ARG1 induction is reduced in a tup1 null mutant strain [13] . However, there is still lack of direct evidence to support this notion, and several studies suggest that Tup1 may continue to act as a corepressor after gene activation. During galactose derepression, for example, the GAL1 gene is induced more quickly in a tup1 null mutant [29] . Similarly, the Drosophila Tup1 orthologue Groucho was recently implicated in transcriptional attenuation of active genes [30] . Here we show that Tup1 facilitates transcriptional deactivation in a manner enhanced by sumoylation. We first demonstrate that Tup1 is sumoylated at two specific lysine residues under various stress conditions. By mutating these sites, we then show that Tup1 sumoylation does not affect its initial recruitment to promoters on activation, but prolongs its association with the promoters, dampens transcription and facilitates eventual removal of RNAP II and the mediator component Gal11. Consistent with this, we identify a Tup1 mutant with enhanced sumoylation that results in reduced transcription. Although sumoylation of Tup1 and Gcn4 has opposite effects on their association with target gene promoters, modification of both proteins results in a net repressive effect on activated transcription. Interestingly, mutation of SUMO sites in both Tup1 and Gcn4 is found to prolong Gcn4 promoter occupancy, suggesting cooperation between sumoylated proteins. These results and others show that Tup1 sumoylation is part of a coordinated SUMO-mediated mechanism of controlling transcription levels and enabling gene deactivation. Tup1 is sumoylated under various stress conditions To extend our studies on the role of sumoylation during gene activation in yeast, we examined how SUMO affects the coactivator/corepressor Tup1. To show that Tup1 is a bona fide SUMO substrate, and to determine whether Tup1 sumoylation is affected by stress conditions, wild-type yeast expressing 6HA-tagged Tup1 (Tup1-HA) in its normal chromosomal location were treated with 100 J m −2 ultraviolet, 1.0 mM H 2 O 2 , nitrogen starvation, carbon starvation, or amino acid starvation (induced by sulfometuron methyl (SM), 0.5 μg ml −1 (ref. 31 )). Tup1-HA was immunoprecipitated (IPed) from cell extracts with an haemagglutinin (HA) antibody and sumoylated forms of Tup1 were detected by Western blot (WB) using an antibody that recognizes yeast SUMO (known as Smt3). We detected sumoylated Tup1-HA from yeast grown in normal, unstressed conditions, but higher levels were found in yeast grown in each of the tested stress conditions ( Fig. 1a ). These results confirm and extend previous global proteomic studies suggesting that Tup1 is a SUMO substrate [14] , [15] , [16] , [17] . Drosophila Groucho is also known to be sumoylated [32] , [33] , suggesting that Tup1 sumoylation is evolutionarily conserved. 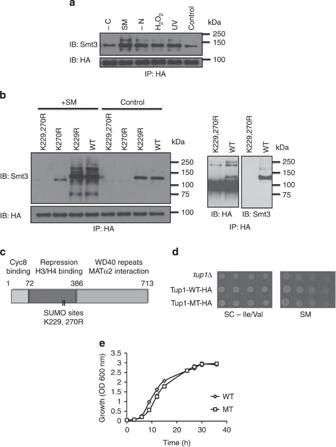Figure 1: Tup1 is sumoylated primarily at K270 with a minor site at K229. (a) HA IPs of untreated cells (control, SC medium), or cells treated with 100 J m−2ultraviolet, H2O2(1.0 mM for 20 min), nitrogen starvation (−N for 60 min), sulfometuron methyl (SM) (0.5 μg ml−1for 20 min) or carbon starvation (−C for 60 min) were analyzed by HA and yeast SUMO (Smt3) immunoblots. (b) Left panel: analysis of HA IPs obtained from untreated control and SM-induced cells expressing either Tup1-6HA WT or mutants plasmids. Right panel: analysis of overexposed HA immunoblot and Smt3 immunoblot of induced cells expressing Tup1-HA-WT and mutant plasmids after HA IP. (c) Diagram of Tup1 protein domains with probable sumoylation sites indicated. (d) Atup1Δstrain was transformed with plasmids expressing either vector, wt Tup1-HA or mutant Tup1-K229,270R. Transformed strains were serially diluted and spotted on medium lacking Val and Ile (left), or the same medium supplemented with 0.5 μg ml−1SM. (e) Growth curve analysis of Tup1-WT and Tup1-MT (K229,270R). Atup1Δstrain was transformed with plasmids expressing either wt Tup1-6HA or mutant Tup1-K229,270R-6HA. Overnight culture were inoculated into fresh SC-Ura medium to OD600of 0.05 and incubated at 30 °C with constant shaking. The absorbance OD600of yeast culture was measured at the indicated time points. Analyses were performed four times, with s.d. indicated with error bars. Figure 1: Tup1 is sumoylated primarily at K270 with a minor site at K229. ( a ) HA IPs of untreated cells (control, SC medium), or cells treated with 100 J m −2 ultraviolet, H 2 O 2 (1.0 mM for 20 min), nitrogen starvation (−N for 60 min), sulfometuron methyl (SM) (0.5 μg ml −1 for 20 min) or carbon starvation (−C for 60 min) were analyzed by HA and yeast SUMO (Smt3) immunoblots. ( b ) Left panel: analysis of HA IPs obtained from untreated control and SM-induced cells expressing either Tup1-6HA WT or mutants plasmids. Right panel: analysis of overexposed HA immunoblot and Smt3 immunoblot of induced cells expressing Tup1-HA-WT and mutant plasmids after HA IP. ( c ) Diagram of Tup1 protein domains with probable sumoylation sites indicated. ( d ) A tup1Δ strain was transformed with plasmids expressing either vector, wt Tup1-HA or mutant Tup1-K229,270R. Transformed strains were serially diluted and spotted on medium lacking Val and Ile (left), or the same medium supplemented with 0.5 μg ml −1 SM. ( e ) Growth curve analysis of Tup1-WT and Tup1-MT (K229,270R). A tup1Δ strain was transformed with plasmids expressing either wt Tup1-6HA or mutant Tup1-K229,270R-6HA. Overnight culture were inoculated into fresh SC-Ura medium to OD 600 of 0.05 and incubated at 30 °C with constant shaking. The absorbance OD 600 of yeast culture was measured at the indicated time points. Analyses were performed four times, with s.d. indicated with error bars. Full size image To facilitate analysis of the function of Tup1 sumoylation, we next mapped its sumoylation site(s). Using the SUMOsp 2.0 sumoylation site prediction programme [34] , three potential sumoylation sites, K229, K270 and K611, were predicted. SUMO WB analysis of Tup1-HA IPs showed multiple bands, which may correspond to sumoylation at multiple sites ( Fig. 1b , left panel). In agreement with this, we found that a single mutation, K270R (see also ref. 17 ), resulted in a major reduction, but not complete loss, of sumoylated Tup1, while another single mutation (K229R) caused a minor reduction after SM treatment. Combining both mutations (K229,270R) almost completely abolished Tup1 sumoylation, implying that K229 and K270 are the sumoylation sites in Tup1, in both untreated and SM-treated cells ( Fig. 1b , left panel). Consistent with this, a minor ~125 kDa form of Tup1-HA, detected when an HA WB was overexposed, was not observed with the K229,270R mutant ( Fig. 1b , right panel). Multiple higher molecular weight forms of Tup1, likely representing further modified isoforms, were also detected in the HA WB (just below the 250 kDa marker; Fig. 1b , right panel), some of which also disappeared with the K229,270R mutations. This indicates that, in addition to sumoylation at K229 and K270, Tup1 is also subject to additional modifications. Unexpectedly, mutation of the third predicted residue, K611, to Arg actually resulted in an increase of sumoylated Tup1 isoforms ( Supplementary Fig. 1a ). While the basis for this is unknown, one explanation is that K611 might normally be subject to other modification(s) that are inhibitory to sumoylation at other Lys residues. Alternatively, mutation of K611 may disrupt protein–protein interactions that naturally limit Tup1 sumoylation at K229 and K270. For example, K611 is located within a WD repeat domain that is capable of binding ubiquitin [35] . The above data indicate that Tup1 is multi-sumoylated (modified by SUMO at multiple Lys residues). To determine whether some sumoylated isoforms were due to poly-sumoylation (SUMO chains forming at single modified Lys residues), we used a strain that expresses a form of Smt3 with Lys-to-Arg mutations at positions thought necessary for chain formation, smt3-R11,15,19 , and another strain in which all Smt3 Lys were mutated to Arg, smt3-allR . These mutants are still capable of conjugating a single SUMO moiety on substrates, but the ability to form polySUMO chains is compromised ( smt3-R11,15,19 ) or abolished ( smt3-allR ) [36] . In WB analysis of Tup1-HA IPs, the signal of sumoylated Tup1 was reduced slightly in the smt3-R11,15,19 mutant, while only a single weak band was detected in the smt3-allR mutant ( Supplementary Fig. 1b ). This result suggests that a significant level of sumoylation associated with Tup1 derives from polySUMO chains. We next set out to investigate phenotypes of mutant yeast strains deficient in Tup1 sumoylation. Since both K229 and K270 sites fall within the central domain which consists of the gene repression, H3/H4 binding and histone deacetylase Hda1 interaction domains [37] , we asked whether sumoylation of Tup1 affects its transcriptional repressive functions ( Fig. 1c ). Notably, Groucho sumoylation sites also fall within the central region required for HDAC interaction, and sumoylation enhances Groucho repressive activity likely through increased interaction with an HDAC [33] . While a tup1 null mutant showed a mild growth defect in SM-containing media [13] , the Tup1-MT (K229,270R) mutant did not show any significant defect when grown on media containing SM ( Fig. 1d ). This result is consistent with the lack of a growth defect of a gcn4 SUMO mutant grown in SM medium [7] . However, analysis of Tup1-WT and Tup1-MT (K229,270R) growth in liquid media revealed a growth delay for Tup1-MT (K229,270R) during exponential phase, although both strains reached the same density during stationary phase ( Fig. 1e ). Taken together, these results suggest that Tup1 sumoylation does not have a general, essential function in Tup1-mediated repression or a direct role in activation of genes induced by amino acid starvation. Tup1 sumoylation enhances repression after gene activation Our previous analyses demonstrated that Smt3 and Ubc9 proteins accumulate at multiple inducible gene promoters during gene activation [6] and that Gcn4 occupancy at target genes can be regulated by sumoylation [7] . To determine whether SUMO-deficient Tup1 also displays altered association with promoters of Gcn4 target genes, we conducted time-course chromatin immunoprecipitation (ChIP) studies of Tup1-HA occupancy in Tup1-WT and Tup1-MT (K229,270R) strains during gene activation induced by SM. 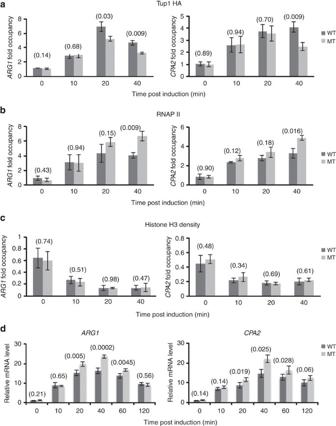Figure 2: Tup1 sumoylation enhances its association with promoters ofARG1andCPA2while reducing their transcription. (a) Tup1-HA ChIP analysis of Tup1 wild-type (WT) or K229,270R mutant (MT) onARG1andCPA2promoters at indicated times after SM induction. (b) RNAP II ChIP analysis of Tup1 wild-type (WT) or K229,270R mutant (MT) onARG1andCPA2promoters at indicated times after SM induction. (c) H3 ChIP analysis of Tup1 wild-type (WT) or K229,270R mutant (MT) onARG1andCPA2promoters at indicated times after SM induction. (d) mRNA levels were determined by RT–PCR forARG1and a control housekeeping gene,ACT1, at the indicated times after exposure to SM. Analysis was performed with strains expressing Tup1-WT or -MT. Values were normalized toARG1RNA levels in Tup1-WT at 0 min. Data are represented as mean±s.d. of three independent experiments.Pvalues (refer to Methods section for calculation) are indicated in parentheses above paired bars where relevant. Figure 2a shows that both Tup1-WT and Tup1-MT (K229,270R) exhibited a similar initial increase in association with the ARG1 and CPA2 promoters after SM treatment. A similar Tup1-WT binding profile on the ARG1 promoter has been previously observed [13] . However, at 20 and 40 min after SM treatment, Tup1-MT (K229,270R) occupancy was significantly lower than Tup1-WT at the ARG1 promoter, while a lower level of Tup1-MT (K229,270R) was detected at the CPA2 promoter at 40 min. A time-course analysis of Tup1-WT sumoylation levels showed that Tup1 sumoylation peaked at 40 min after SM treatment, indicating that the greatest differential in Tup1-WT versus Tup1-MT (K229,270R) promoter occupancy was observed when Tup1 is normally most highly sumoylated ( Supplementary Fig. 1c ). To determine whether Tup1 associates specifically with promoter regions, we performed ChIP of Tup1-HA on the ARG1 promoter, coding and downstream untranscribed regions ( Supplementary Fig. 2a ). We detected both Tup1-WT and Tup1-MT (K229,270R) mostly on the promoter region, and only after SM treatment, suggesting that Tup1 indeed associates with inducible gene promoter regions. Figure 2: Tup1 sumoylation enhances its association with promoters of ARG1 and CPA2 while reducing their transcription. ( a ) Tup1-HA ChIP analysis of Tup1 wild-type (WT) or K229,270R mutant (MT) on ARG1 and CPA2 promoters at indicated times after SM induction. ( b ) RNAP II ChIP analysis of Tup1 wild-type (WT) or K229,270R mutant (MT) on ARG1 and CPA2 promoters at indicated times after SM induction. ( c ) H3 ChIP analysis of Tup1 wild-type (WT) or K229,270R mutant (MT) on ARG1 and CPA2 promoters at indicated times after SM induction. ( d ) mRNA levels were determined by RT–PCR for ARG1 and a control housekeeping gene, ACT1 , at the indicated times after exposure to SM. Analysis was performed with strains expressing Tup1-WT or -MT. Values were normalized to ARG1 RNA levels in Tup1-WT at 0 min. Data are represented as mean±s.d. of three independent experiments. P values (refer to Methods section for calculation) are indicated in parentheses above paired bars where relevant. Full size image To extend these results, we examined Tup1-WT and Tup1-MT (K229,270R) promoter occupancy on two additional Tup1 target genes, HIS4 and SUC2 . The HIS4 gene is also responsive to SM treatment [31] , and time-course ChIP ( Supplementary Fig. 2b ) revealed profiles for both Tup1 derivatives very similar to those observed with the ARG1 and CPA2 promoters, that is, reduced Tup1-MT (K229,270R) occupancy at later times. In contrast, the SUC2 promoter is responsive to low glucose starvation, but not to SM treatment, and no differences in Tup1-WT and Tup1-MT (K229,270R) occupancy were detected ( Supplementary Fig. 2c ). These results suggest that the effect of Tup1 sumoylation on Tup1 target genes is not universal and perhaps condition dependent. Reduced Tup1-MT (K229,270R) on SM-inducible target promoters was not due to lower expression levels of the mutant protein. On the contrary, in many cases, especially when strains were grown in nutrient-poor media, such as in the presence of proline as the main source of nitrogen, we detected significantly higher levels of Tup1-MT (K229,270R) than Tup1-WT ( Supplementary Fig. 3a ), suggesting that Tup1 sumoylation is involved in promoting Tup1 degradation. Similarly, sumoylation of Drosophila Groucho also promotes its degradation, via an ubiquitin-mediated pathway [32] . However, deletion of genes encoding SUMO-targeted ubiquitin ligases Slx5 or Rad18 did not result in increased Tup1-HA levels in cells grown under standard conditions, suggesting that sumoylation of Tup1 does not normally trigger its degradation through a ubiquitin pathway ( Supplementary Fig. 3b ). Together, our results indicate that Tup1 is recruited to target gene promoters during activation independent of sumoylation, but preventing its sumoylation can, in a gene- and/or condition-dependent manner, result in lower occupancy at later time points. In light of the above results, we next examined whether Tup1 sumoylation affects recruitment of RNAP II to the ARG1 and CPA2 promoters, again by time-course ChIP during SM induction. As with Tup1 itself, we did not observe any difference in RNAP II levels between Tup1-WT and Tup1-MT (K229,270R) strains at the beginning of the time course. However, increased levels of RNAP II were detected at both promoters in the Tup1-MT (K229,270R) strain at the 40-min time point ( Fig. 2b ). This is consistent with the reduced levels of promoter-associated Tup1-MT (K229,270R) allowing increased RNAP II recruitment. Conditional removal of Tup1 was previously shown to cause decreased histone H3 occupancy at several promoters [26] , and it was thus conceivable that defective Tup1 sumoylation might have a similar effect. We therefore compared histone H3 levels at the above promoters in Tup1-WT and Tup1-MT (K229,270R) strains during induction. In both strains, H3 levels dropped during the time course, reflecting gene activation, but we detected no difference in H3 occupancy between the two strains ( Fig. 2c ). Together, these results indicate that sumoylation regulates Tup1 occupancy on target gene promoters, as we observed previously with Gcn4 (ref. 7 ). However, while blocking Gcn4 sumoylation resulted in increased Gcn4 promoter occupancy, blocking Tup1 sumoylation had the opposite effect, causing reduced Tup1 persistence as well as increased RNAP II recruitment, which was not due to secondary effects on histone H3 levels. To determine whether the reduced binding of SUMO-deficient Tup1 affects target gene expression, we performed reverse transcription quantitative PCR analysis of ARG1 and CPA2 transcripts over a time course after SM treatment with the Tup1-WT and Tup1-MT (K229,270R) strains ( Fig. 2d ). The messenger RNA (mRNA) levels of ARG1 and CPA2 peaked at the 40-min time point and decreased gradually at the 60 and 120 min time points. Similar to the ChIP analysis, we did not detect any significant initial difference in ARG1 and CPA2 mRNA levels between WT and MT (K229,270R) (first 10 min after SM treatment). However, both ARG1 and CPA2 mRNA levels were significantly higher in the Tup1-MT (K229,270R) strain at the 20, 40 and 60 min time points, correlating well with our observation that less Tup1-MT (K229,270R), and more RNAP II, was present at these promoters at later points during the time course. Strengthening these findings, we also found that a strain expressing the hyper-sumoylated Tup1 mutant (K611R) generated reduced ARG1 mRNA levels compared with a WT strain ( Supplementary Fig. 4 ). Taken together, our findings demonstrate that Tup1 sumoylation can affect target gene transcription in a negative manner, indicating a role in modulating, or dampening, activated transcription. Tup1 and Gcn4 sumoylation modulates Gcn4 promoter binding Recent studies suggest that sumoylation can coordinately regulate multiple components of protein complexes, as opposed to regulating individual proteins independently, to achieve a biological effect. Consequently, stronger effects can be detected when sumoylation of several SUMO targets in the same complex is blocked [38] , [39] . In light of this, we examined the effect of combining SUMO site mutations in both Tup1 and Gcn4. Strains expressing either chromosomally tagged Tup1-WT or Tup1-K270R were generated and transformed with either Gcn4-WT or Gcn4 SUMO-deficient mutant (K50,58R) expression plasmids. Time-course ChIP analyses of Gcn4-Flag showed that the Tup1 SUMO mutation on its own slightly enhanced Gcn4-WT occupancy at the ARG1 promoter following SM treatment ( Fig. 3a ). As we previously observed [7] , mutation of Gcn4 SUMO sites also resulted in increased Gcn4 occupancy on the ARG1 promoter. Interestingly though, simultaneous mutation of SUMO sites on Tup1 and Gcn4 resulted in a considerably greater increase in Gcn4 promoter occupancy after SM treatment ( Fig. 3a ). Although individual SUMO site mutations on both Tup1 and Gcn4 resulted in increased ARG1 transcript levels, combining the mutations did not result in a further increase ( Fig. 3b ), perhaps because maximal activation rates had already been achieved. These results nonetheless indicate that Tup1 sumoylation can affect promoter levels of Gcn4, and suggest that coordinated sumoylation of Tup1 and Gcn4, and possibly other promoter-bound factors (see below), ensures efficient clearance of Gcn4 from target genes. 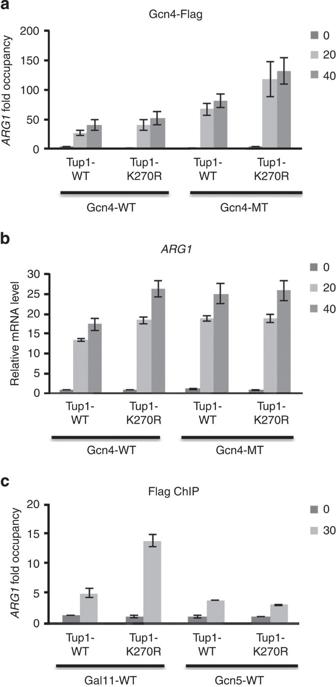Figure 3: Sumoylation of both Tup1 and Gcn4 enhances Gcn4 eviction from the inducedARG1promoter. (a) Gcn4-Flag WT and K50,58R MT ChIP analysis of Tup1 wild-type (WT) or K270R mutant onARG1promoter at indicated times after SM induction. (b) mRNA levels were determined by RT–PCR forARG1andACT1at the indicated times after exposure to SM. Analysis was performed in strains expressing Gcn4-WT or K50,58R (MT) and Tup1-WT, or K270R, as indicated. Values were normalized toARG1mRNA levels in strain expressing Gcn4-WT and Tup1-WT at 0 min. (c) Gal11-WT and Gcn5-WT Flag ChIP analysis of Tup1 wild-type (WT) or K270R mutant onARG1promoters at indicated times after SM induction. Data are represented as mean±s.d. of three independent experiments. Figure 3: Sumoylation of both Tup1 and Gcn4 enhances Gcn4 eviction from the induced ARG1 promoter. ( a ) Gcn4-Flag WT and K50,58R MT ChIP analysis of Tup1 wild-type (WT) or K270R mutant on ARG1 promoter at indicated times after SM induction. ( b ) mRNA levels were determined by RT–PCR for ARG1 and ACT1 at the indicated times after exposure to SM. Analysis was performed in strains expressing Gcn4-WT or K50,58R (MT) and Tup1-WT, or K270R, as indicated. Values were normalized to ARG1 mRNA levels in strain expressing Gcn4-WT and Tup1-WT at 0 min. ( c ) Gal11-WT and Gcn5-WT Flag ChIP analysis of Tup1 wild-type (WT) or K270R mutant on ARG1 promoters at indicated times after SM induction. Data are represented as mean±s.d. of three independent experiments. Full size image Sumoylated Tup1 impairs recruitment of Gal11 but not Gcn5 We next wished to determine whether the repressive effect of Tup1 sumoylation involves additional proteins that function in ARG1 activation. In addition to Tup1 and Gcn4, Gal11 and Gcn5 have been identified as SUMO targets [14] , [16] , [40] . Gcn4 interacts with Gal11 directly, and this interaction is important for efficient Gal11 recruitment to the ARG1 promoter [41] . Moreover, depletion of Tup1 caused a significant increase in occupancy of both Gal11 and Gcn5 at several promoters [26] . We therefore investigated whether the repressive effect of sumoylated Tup1 reflects effects on binding of Gal11 and/or Gcn5. Strains expressing different combinations of chromosomally Tup1-HA-WT or Tup1-K270R and Flag-tagged Gcn5-WT or Gal11-WT were generated. ChIP analysis confirmed that induction of ARG1 by SM coincided with recruitment of both Gal11 and Gcn5 to the ARG1 promoter ( Fig. 3c ). While Gcn5-Flag occupancy was unaffected by the Tup1 SUMO site mutations, sharply elevated levels of Gal11-Flag were detected at the ARG1 promoter in the Tup1-K270R strain. The magnitude of the effect (approximately threefold) was significantly higher than the effect of Tup1 mutation on its own occupancy (~30% reduction in Tup1 occupancy; compare Figs 3c and 2a ), indicating that increased Gal11 levels were not simply a consequence of reduced Tup1 on the promoter. This result is consistent with our findings that impaired Tup1 sumoylation resulted in higher levels of RNAP II at the ARG1 promoter. Taken together, our data point to a coordinated effect of Tup1 sumoylation on the ARG1 promoter that enhances deactivation of activated transcription. Tup1-interacting factors are sumoylated after SM treatment We next wished to investigate further the possibility that the effect of Tup1 sumoylation on promoter deactivation involves a coordinated network of sumoylated proteins, that is, a consequence of ‘protein-group sumoylation’ [39] . To this end, we examined whether other proteins known to interact physically or genetically with Tup1 are also SUMO targets, and whether their sumoylation is induced by SM treatment. These include histone H3 (ref. 42 ), Cti6, which relieves Tup1 transcriptional repression [25] , Gcn5 (ref. 43 ), Gal11 (refs 24 , 26 ) and Cyc8 (refs 20 , 44 , 45 ). We generated strains expressing HA-tagged versions of each of these proteins from their chromosomal loci, and subjected them to SM treatment for 20 min. The HA-tagged proteins were IPed from whole-cell extracts and analyzed by SUMO WB. In every case, we detected sumoylation of the tested protein in untreated cells, but SM treatment resulted in significantly higher levels of sumoylation ( Fig. 4a ). This indicates that Tup1-associated proteins are coordinately sumoylated on induction of target genes. This did not reflect a global increase in sumoylation induced by SM, as analysis of whole-cell lysates, prepared from three different yeast strains, by SUMO WB revealed at most very slight increases in total sumoylation after SM treatment ( Supplementary Fig. 5a ), suggesting that the increase in sumoylation of Tup1-associated proteins was part of a specific response during gene activation by SM. Supporting this conclusion, we observed no increase in sumoylation of Tfg1, a subunit of transcription factor TFIIF, after SM treatment ( Supplementary Fig. 5b ), even though Tfg1 is a known SUMO target [14] , [15] , [16] . 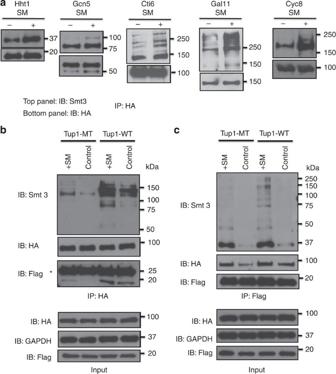Figure 4: Multiple Tup1- and transcription-related proteins are sumoylated during amino acid starvation. (a) Hht1-HA, Gcn5-HA, Cti6-HA, Gal11-HA and Cyc8-HA IPs of untreated (control), or SM-treated cells were analyzed by HA and yeast SUMO (Smt3) Western blots. (b) Analysis of HA IPs obtained from untreated control and SM-induced cells expressing Hht1-WT Flag and either Tup1-WT-HA or K270R-HA. The asterisk indicates the HA antibody light chain. (c) Analysis of Flag IPs obtained from untreated control and SM-induced cells expressing Hht1-WT Flag and either Tup1-WT-HA or K270R-HA. Figure 4: Multiple Tup1- and transcription-related proteins are sumoylated during amino acid starvation. ( a ) Hht1-HA, Gcn5-HA, Cti6-HA, Gal11-HA and Cyc8-HA IPs of untreated (control), or SM-treated cells were analyzed by HA and yeast SUMO (Smt3) Western blots. ( b ) Analysis of HA IPs obtained from untreated control and SM-induced cells expressing Hht1-WT Flag and either Tup1-WT-HA or K270R-HA. The asterisk indicates the HA antibody light chain. ( c ) Analysis of Flag IPs obtained from untreated control and SM-induced cells expressing Hht1-WT Flag and either Tup1-WT-HA or K270R-HA. Full size image Gcn5 and histone H3 have previously been identified as SUMO substrates, and both sumoylated forms play negative roles in transcription regulation [40] , [46] . More recently, desumoylation of Cyc8 has been implicated in derepression of GAL1 transcription [8] . In studies mentioned above, DNA damage was shown to induce sumoylation of multiple proteins involved in the DNA repair pathway, creating a synergistic response to DNA damage and promoting protein–protein interactions [38] , [39] . Likewise, we suggest that simultaneous sumoylation of Tup1, Gcn4 and associated proteins during gene activation functions to ensure subsequent transcriptional deactivation. We next wished to investigate whether Tup1 sumoylation affects interactions with any of its network of associated factors. To this end, we examined whether sumoylation of Tup1 affects its association with histone H3. Reciprocal co-IP experiments with strains expressing Flag-tagged Hht1 (histone H3) and either Tup1-HA-WT or Tup1-MT (K270R) were performed. Tup1-HA was IPed from whole-cell extracts with an HA antibody, and sumoylated forms of Tup1 and co-IPed Flag-Hht1 were detected by WB using an Smt3 antibody and an Flag antibody, respectively ( Fig. 4b ). We detected increased association of Flag-Hht1 with Tup1-WT after SM treatment. However, association was strongly reduced in the Tup1-MT strain. Similarly, in the reciprocal Flag IP more Tup1-WT than Tup1-MT co-IPed with Flag-Hht1 after SM treatment ( Fig. 4c ). These results indicate that Tup1 sumoylation enhances its interaction with H3, likely contributing to Tup1-mediated gene deactivation. Interestingly, a Smt3 WB of the Flag-Hht1 IP revealed fewer sumoylated species associated with Hht1 when Tup1 sumoylation was impaired ( Fig. 4c ). This supports the idea that Tup1 sumoylation is important for coordinating SUMO modifications of additional components of Tup1/Hht1-containing complexes. Transcription initiation by RNAP II is an immensely complex process involving numerous multi-subunit protein factors. While the molecular mechanisms of inducible gene activation following stimulation are well-characterized, it has been much less clear how transcription is returned to basal levels, or how genes are shut off, following activation. Our previous analyses demonstrated that sumoylation of Gcn4 is required for its efficient removal from promoters following transcription activation [7] , and similar findings with the mammalian activator AP-1 suggest this mechanism is evolutionarily conserved [9] . However, removal or inactivation of an activator can be insufficient to stop transcription entirely or to return a gene to an inactive state, and indeed Tup1 becomes ineffective under such conditions [47] . Thus, while our data have established important roles for SUMO-mediated clearance of Gcn4 and stabilization of Tup1 binding in promoter deactivation, additional mechanisms must be at play to insure efficient deactivation of induced genes when their products are no longer needed. Our results showing that multiple Tup1-associated proteins display enhanced sumoylation on induction point to a role for a ‘protein-group’ sumoylation mechanism, as has been observed for several other nuclear processes involving complex protein assemblies [39] . As we have previously observed promoter-associated sumoylation during induction of other types of genes, such as GAL1 and STL1 (ref. 6 ), we suggest that sumoylation of distinct protein complexes found on different activated promoters is a general mechanism of regulating transcription. In any event, our study has demonstrated that sumoylation plays an important role in fine-tuning gene expression during activation and subsequent deactivation, and that SUMO-dependent modulation of Tup1 repression activity plays an important role in this process Yeast strains and plasmids All yeast strains used are listed in Supplementary Table 1 . The chromosomally 6HA- and 3HA-tagged yeast strains (CHNM1 to 8 and YAA set) were generated by homologous recombination under the selection of minimal media without tryptophan [48] . The presence of the tagged alleles was verified by colony PCR and WB analysis using anti-HA antibodies. The pTUP1-6HA plasmid was generated by first amplifying TUP1 genomic DNA including 1 kb upstream and downstream of the TUP1 ORF and subsequently cloning the PCR product using the URA3 -marked CEN vector pRS316. For generation of integrative mutagenic alleles, a site-directed mutagenesis PCR-based homologous recombination approach was employed [49] , while for generation of the mutagenic plasmid, a highly efficient site-directed, ligase-independent mutagenesis approach was used [50] . The details of the cloning procedure are available on request. Primer sequences are listed in Supplementary Table 2 . WB and IP Yeast cultures were grown in minimal medium lacking isoleucine and valine at OD 600 of 0.6–0.7. Induction of Tup1 target genes, ARG1 and CPA2 by amino acid starvation was achieved by treatment with SM from Sigma at a final concentration of 0.5 μg ml −1 for 20 min (unless otherwise specified). Cells were lysed by agitation with glass beads in IP buffer (150 mM NaCl, 50 mM Tris pH 8.0, 0.1% NP-40 and 10% glycerol) plus 2.5 mg ml −1 N-ethylmaleimide. IPs and washes were performed in the same buffer, and 1 μg of the appropriate antibody was added for overnight IP with Protein-G-sepharose beads. Proteasomal inhibition [51] was performed by addition of 20 μM MG132 or mock treatment (DMSO) for 1 h before harvesting for WB analysis. Chromatin immunoprecipitation (ChIP) Exponentially growing yeast were treated (as indicated in Fig. 1a ), or mock treated, then cross-linked with 1% formaldehyde for 20 min, before quenching with 0.36 M glycine. Samples were pelleted by centrifugation and washed once with ice-cold TBS (20 mM Tris-HCl, pH 7.5 and 150 mM NaCl), then in ChIP buffer (0.05 M HEPES-KOH, pH 7.5, 150 mM NaCl, 1 mM EDTA, 1% Triton X-100, 0.1% sodium deoxycholate and 0.1% SDS). Pelleted samples were re-supsended in 600 μl of ChIP buffer and 400 μl of glass beads were added before they were subjected to three rounds of 1-min bead beating, with 1-min breaks in between. Lysates were recovered and sonicated to shear chromatin into fragments with an average length of ~500 bp. Samples were then microcentrifuged and NaCl was added to the supernatants to adjust the final concentration to 275 mM. IPs were then performed overnight, with 1 μg of appropriate antibody and Protein G-sepharose beads added to the samples. Beads were then washed first in ChIP buffer with 275 mM NaCl, then in ChIP buffer with 500 mM NaCl, then in an additional wash buffer (10 mM Tris-HCl, pH 8, 0.25 M LiCl, 1 mM EDTA, 0.5% NP-40 and 0.5% sodium deoxycholate) and finally in Tris-EDTA buffer buffer (10 mM Tris-HCl, pH 8 and 1 mM EDTA). IPed chromatin was eluted by incubation of beads in ChIP Elution Buffer (50 mM Tris-HCl, pH 7.5, 10 mM EDTA and 1% SDS) at 65 °C for 10 min. Samples were microcentrifuged and the supernatant was treated with proteinase K for 1 h at 42 °C, before cross-links were reversed by heating to 65 °C for at least 4 h. DNA was recovered by phenol–chloroform extraction and ethanol precipitation, then analyzed by PCR. Primer sequences are listed in Supplementary Table 2 . For quantification, a two-tailed Student’s t -test was applied with P values indicated in parentheses above paired bars within graphs for statistical data analysis. Antibodies Antibodies used for WB, IP and ChIP assay were anti-Flag M2 (Sigma, cat. F1804, WB—1:1,000), rabbit anti-HA (abm, cat. G166, WB—1:1,000), mouse anti-HA (Covance, cat. MMS101P, WB—1:1,000), rabbit anti-H3 (abm, cat. ab1791, WB—1:2,000), anti-GADPH (Sigma, cat. G9545, WB—1:2,000), rabbit anti-Smt3 (Santa Cruz, cat. sc-28649, WB—1:1,000) and rabbit anti-Rpb1 (Santa Cruz, cat. sc-25758). The uncropped scans of the Figs 1a,b and 4a–c are included in Supplementary Fig. 6 . Quantitative real time PCR was performed using gene-specific primers and the primer sequences are listed in Supplementary Table 2 . How to cite this article: Ng, C. H. et al . Sumoylation controls the timing of Tup1-mediated transcriptional deactivation. Nat. Commun , 6:6610 doi: 10.1038/ncomms7610 (2015).